Phase fluctuations and the absence of topological defects in a photo-excited charge-ordered nickelate The dynamics of an order parameter's amplitude and phase determines the collective behaviour of novel states emerging in complex materials. Time- and momentum-resolved pump-probe spectroscopy, by virtue of measuring material properties at atomic and electronic time scales out of equilibrium, can decouple entangled degrees of freedom by visualizing their corresponding dynamics in the time domain. Here we combine time-resolved femotosecond optical and resonant X-ray diffraction measurements on charge ordered La 1.75 Sr 0.25 NiO 4 to reveal unforeseen photoinduced phase fluctuations of the charge order parameter. Such fluctuations preserve long-range order without creating topological defects, distinct from thermal phase fluctuations near the critical temperature in equilibrium. Importantly, relaxation of the phase fluctuations is found to be an order of magnitude slower than that of the order parameter's amplitude fluctuations, and thus limits charge order recovery. This new aspect of phase fluctuations provides a more holistic view of the phase's importance in ordering phenomena of quantum matter. The central question of strongly correlated materials is the emergence of symmetry-breaking novel quantum states, such as high-temperature superconductivity, charge-, spin- and orbital-ordering states [1] . Recently, an increasing number of experiments have demonstrated the possibility of manipulating this emergence using ultrafast light sources to create novel transient states that are inaccessible from thermal equilibrium [2] , [3] , [4] . Deciphering the underlying charge [5] , [6] , spin [7] , [8] and lattice dynamics [9] , and particularly collective behaviours of emergent novel quantum states [10] , [11] , [12] , holds the key to uncovering mysteries of these photoinduced phenomena. As the collective properties of many of these symmetry-breaking novel quantum states can be described by a complex order parameter, consisting of an amplitude and phase, it is crucial to directly measure the dynamics of order parameters' amplitude and phase in these photoinduced transient states. To demonstrate such photoinduced dynamics of a long-rang order parameter, we take the charge order (CO) in striped nickelate as an example. Using femtosecond resonant X-ray diffraction (RXD), the dynamics of the CO order parameter can be directly monitored. Despite dramatic suppression of the CO diffraction peak intensity, both the CO period and correlation length are essentially unchanged up to 25 ps after the pump laser excitation. Furthermore, we identify the unforeseen photoinduced phase fluctuations of the CO order parameter, which relaxes at a much slower timescale than the recovery of the CO amplitude. Our results demonstrate the importance of the order parameter's phase fluctuation that is not only important in determining thermodynamics in equilibrium but also crucial in the emergence of such novel quantum states under non-equilibrium conditions. Striped nickelate and RXD In striped nickelates, charge and spin order (SO) coexist at low temperatures, where doped charge carriers form one-dimensional charge density waves, and spins align in spin density waves with half the CO period ( Fig. 1a ) [13] , [14] , [15] , [16] , [17] , [18] . The CO order parameter's amplitude is related to the periodic valence difference of Ni 2+ and Ni 3+ ions and the order parameter's phase is the angle characterizing the periodic function of the CO, which is a constant when CO is uniformly ordered. Similar stripe phases also have been found in doped cuprates [19] , [20] , where they are thought to compete against high-temperature superconductivity. In the present work, both time-resolved optical reflectivity and RXD [21] were used to reveal the dynamics of the CO order parameter. Whereas time-resolved optical reflectivity measurements reveal local charge dynamics, RXD is directly sensitive to the long-range correlation of CO. Owing to significant resonance effects at the Ni L-edge (2 p -3 d transition), the RXD signal at the CO wavevector is dominated by the Bragg scattering from the valence electron modulation of Ni ions [17] ; the contribution of photon scattering from associated periodic lattice distortion is negligible. The RXD intensity can be expressed as |Δ| 2 e - w phase , which is proportional to the CO order parameter's amplitude (Δ) and a Debye–Waller-like factor ( w phase ) due to phase fluctuation of the electronic CO [22] , [23] , [24] , which is essentially the vibration of the electronic CO. In addition, the correlation length of CO can be inferred from the width of the CO diffraction peak. Therefore, time-resolved RXD is an ideal probe to measure the dynamics of electronic CO order parameters. Only recently, time-resolved RXD with femtosecond resolution ( Fig. 1b ) has become possible owing to the recently commissioned femtosecond X-ray free electron laser (FEL) at the Linac Coherent Light Source [25] . A single bright X-ray FEL pulse can generate analyzable diffraction patterns for CO ( Fig. 1c ), allowing pulse-by-pulse data acquisition for correcting the X-ray FEL timing and intensity jitter in the data analysis. The overall temporal resolution is ~0.4 ps limited by the synchronization between the pump laser and X-ray FEL pulse [26] . Details of the experimental set-up are described in the Methods. 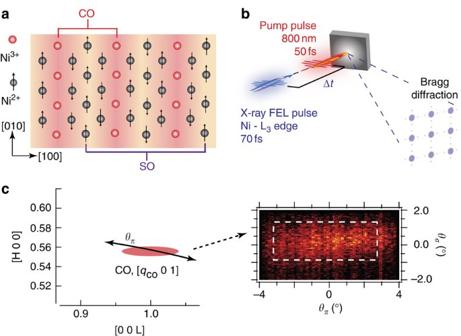Figure 1: Striped nickelate. (a) A cartoon of the stripe state in doped nickelate with doping levelx=0.25. In this simplified ionic cartoon picture, doped holes mostly reside on Ni3+ions, whereas the remaining Ni2+ions are at high-spin state (S=1). CO labels the charge order where one dimensional charge (Ni3+) stripes arrange periodically, serving as anti-phase domain walls for antiferromagnetically ordered spin (Ni2+) stripes (labelled as SO). (b) A sketch of the optical pump and RXD-resonant diffraction probe experiment. At time zero (Δt=0), the sample was pumped by an optical laser pulse (800 nm, 50 fs); an X-ray free electron laser (FEL) probe pulse with a temporal duration less than 70 fs was introduced at a time delay Δtto map out the time evolution of the CO-resonant diffraction peaks. (c) Reciprocal space diagram for the locations of the CO diffraction peaks, whereqco~0.554 (2π/a) for the measured sample. Orthorhombic notation14is used to express the position of the SO and CO in the reciprocal space. Also shown are the CO diffraction peaks captured by a fast CCD detector16. The diffraction peak images are produced by a single X-ray FEL pulse tuned to 851 eV, corresponding to the Ni L3-edge (2p– 3dtransition). The horizontal axis (θπ) of the image is parallel to the scattering plane, corresponding to the cut (black solid curve) through the diffraction peak in the [H 0 L] plane. The vertical axisθσσis perpendicular to the scattering plane, corresponding to the [0 K 0] direction. The white box indicates the region used to calculate integrated intensity of CO diffraction peak. Figure 1: Striped nickelate. ( a ) A cartoon of the stripe state in doped nickelate with doping level x =0.25. In this simplified ionic cartoon picture, doped holes mostly reside on Ni 3+ ions, whereas the remaining Ni 2+ ions are at high-spin state ( S =1). CO labels the charge order where one dimensional charge (Ni 3+ ) stripes arrange periodically, serving as anti-phase domain walls for antiferromagnetically ordered spin (Ni 2+ ) stripes (labelled as SO). ( b ) A sketch of the optical pump and RXD-resonant diffraction probe experiment. At time zero (Δ t =0), the sample was pumped by an optical laser pulse (800 nm, 50 fs); an X-ray free electron laser (FEL) probe pulse with a temporal duration less than 70 fs was introduced at a time delay Δ t to map out the time evolution of the CO-resonant diffraction peaks. ( c ) Reciprocal space diagram for the locations of the CO diffraction peaks, where q co ~0.554 (2π/ a ) for the measured sample. Orthorhombic notation [14] is used to express the position of the SO and CO in the reciprocal space. Also shown are the CO diffraction peaks captured by a fast CCD detector [16] . The diffraction peak images are produced by a single X-ray FEL pulse tuned to 851 eV, corresponding to the Ni L 3 -edge (2 p – 3 d transition). The horizontal axis ( θ π ) of the image is parallel to the scattering plane, corresponding to the cut (black solid curve) through the diffraction peak in the [H 0 L] plane. The vertical axis θσ σ is perpendicular to the scattering plane, corresponding to the [0 K 0] direction. The white box indicates the region used to calculate integrated intensity of CO diffraction peak. 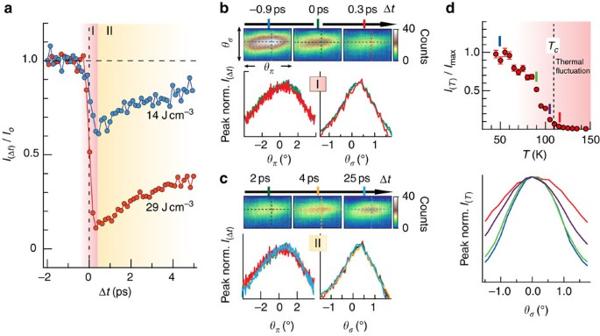Figure 2: Early dynamics of the charge order. (a) Integrated intensity of CO diffraction peak plotted within the first 5 ps after time zero. The pump excitation density is indicated by associated labels. The data shown here were taken at 50 K. (b,c) Evolution of the CO peak at the excitation density of 29 J cm−3in regions I (b) and II (c). Images at representative time delays were obtained from an average of approximately 30–40 X-ray FEL pulses. Colour scale on the side of the images indicates corresponding counts on the detector. Below the images, peak-intensity-normalized line cuts along the colour-coded dashed lines are plotted with associated colours corresponding to colour-coded ticks at representative time delays. (d) Temperature dependence of the CO-resonant diffraction peak measured in thermal equilibrium conditions at a synchrotron light source. The peak intensities are plotted in the upper panel. The red-shaded area indicates the temperature range where the thermal fluctuation is significant. Lower panel displays peak-intensity-normalized line cuts alongθσat representative temperatures, as indicated by colour ticks in the upper panel. Full size image Evolution of CO order parameter Figure 2a shows the early dynamics of the integrated intensity of the CO diffraction peak for two different pump excitation densities. Following the optical pump pulse at time zero, the intensity drops sharply (region I), indicating a photoinduced suppression of CO, likely due to inter-site transitions between Ni ions caused by absorbing 800 nm pump photons [27] . After reaching a minimum, the intensity recovers toward its original value (region II). Figure 2b,c displays the evolution of the CO diffraction peak for a given excitation density. Within our experimental accuracy, no variation of the peak position can be resolved in either region I or II, indicating that the period of CO essentially remains unchanged in the photo-excited transient state. Importantly, the width of the CO peak shows no sign of broadening in the investigated time range, suggesting that the correlation length does not shorten due to photo excitation despite a significant reduction in the peak intensity. This is in sharp contrast to thermal evolution of the CO diffraction peak near the equilibrium phase transition temperature where a suppression of the peak intensity to a similar level (for example, T =105 K) is accompanied by width broadening [14] , [15] , [16] ( Fig. 2c ) due to the creation of topological defects [28] in CO. Thus, in the photoinduced non-equilibrium state, CO peak intensity can vary dramatically without changing the CO length scales. Figure 2: Early dynamics of the charge order. ( a ) Integrated intensity of CO diffraction peak plotted within the first 5 ps after time zero. The pump excitation density is indicated by associated labels. The data shown here were taken at 50 K. ( b , c ) Evolution of the CO peak at the excitation density of 29 J cm −3 in regions I ( b ) and II ( c ). Images at representative time delays were obtained from an average of approximately 30–40 X-ray FEL pulses. Colour scale on the side of the images indicates corresponding counts on the detector. Below the images, peak-intensity-normalized line cuts along the colour-coded dashed lines are plotted with associated colours corresponding to colour-coded ticks at representative time delays. ( d ) Temperature dependence of the CO-resonant diffraction peak measured in thermal equilibrium conditions at a synchrotron light source. The peak intensities are plotted in the upper panel. The red-shaded area indicates the temperature range where the thermal fluctuation is significant. Lower panel displays peak-intensity-normalized line cuts along θ σ at representative temperatures, as indicated by colour ticks in the upper panel. Full size image Recovery timescales The timescales exhibited in the recovery reveal further information about the CO dynamics. As demonstrated in Fig. 3a , the recovery of CO peak intensity (up to Δ t =25 ps) is characterized by two recovery processes with distinct timescales, ~2 ps and ~60 ps, varying by more than one order of magnitude ( Supplementary Methods ). Furthermore, the component of the slower dynamics is significant, because it limits the recovery of the CO peak intensity. To gain further insight into the origin of these two timescales, it is informative to compare RXD data with optical reflectivity data, which is sensitive to the local charge dynamics [5] , [6] . The recovery of photoinduced reflectivity change Δ R/R ( Fig. 3b ) is similarly characterized by two recovery processes: a faster and dominant component of ~0.5 ps, plus a slower recovery of ~2 ps. Comparing the timescales deduced from the two techniques, we find that is similar to ; however, the dynamics corresponding to and are not evident in the optical reflectivity and RXD data, respectively. These observations are further confirmed by the pump excitation dependence summarized in Fig. 3c . Clearly, three different dynamics are involved, and both and are similar within the range of investigated pump excitation density. Also, increases more pronouncedly than the other two timescales, as the pump excitation density increases, implying a different origin than that of for long-range CO recovery. 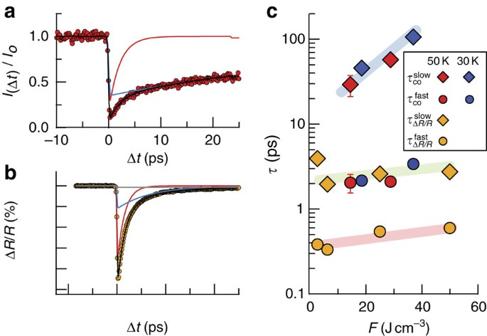Figure 3: Comparison of recovery timescales. (a) Time-dependent integrated intensity of the CO diffraction peak, which was fitted with two exponential functions. Red and blue curves are the fitted fast (2 ps) and slow dynamics (57 ps), respectively. The black curve is the corresponding best fit to the data. (b) Time-dependent reflectivity change ΔR/Rat a wavelength of 800 nm. The time traces were fitted with a fast (red curve, 0.5 ps) and slow (blue curve, 2.7 ps) exponential recovery in addition to a constant background (grey curve), representing a long-living meta-stable state in the local charge channel. The black curve is the corresponding best fit to the data. (c) Fast and slow recovery timescales deduced from the integrated intensity of CO (τCO) and optical ΔR/Rdata (τΔR/R). No difference can be discerned between the dynamics measured at 30 K and 50 K. The red-, green- and blue-shaded areas are guides-to-the-eye for the three dynamics deduced from both CO diffraction peak and ΔR/Rdata. Temporal resolution was taken into account as a Gaussian convolution in the fitting processes. The error bars are determined by 95% confidence interval of the fit. Figure 3: Comparison of recovery timescales. ( a ) Time-dependent integrated intensity of the CO diffraction peak, which was fitted with two exponential functions. Red and blue curves are the fitted fast (2 ps) and slow dynamics (57 ps), respectively. The black curve is the corresponding best fit to the data. ( b ) Time-dependent reflectivity change Δ R/R at a wavelength of 800 nm. The time traces were fitted with a fast (red curve, 0.5 ps) and slow (blue curve, 2.7 ps) exponential recovery in addition to a constant background (grey curve), representing a long-living meta-stable state in the local charge channel. The black curve is the corresponding best fit to the data. ( c ) Fast and slow recovery timescales deduced from the integrated intensity of CO ( τ CO ) and optical Δ R/R data ( τ Δ R / R ). No difference can be discerned between the dynamics measured at 30 K and 50 K. The red-, green- and blue-shaded areas are guides-to-the-eye for the three dynamics deduced from both CO diffraction peak and Δ R/R data. Temporal resolution was taken into account as a Gaussian convolution in the fitting processes. The error bars are determined by 95% confidence interval of the fit. Full size image We note that Eichberger et al . [10] have reported a similar observation by comparing recovery timescales of optical reflectivity to those of femtosecond electron diffraction in TaS 2 . As femtosecond electron diffraction is only sensitive to atomic positions, the distinct timescales have been attributed to the distinction between electronic and lattice order parameters. In contrast, our time-resolved RXD measurements provide hereto unforeseen behaviour of the electronic order parameter dynamics, as the CO diffraction peak at the Ni L 3 -edge in striped nickelates is dominated by light scattered by the Ni valence electron density modulation [17] , whereas the contribution of the scattering from associated periodic lattice distortion is negligible. Therefore, the recovery timescales deduced from the optical reflectivity and RXD are all of electronic origin, but correspond to three different dynamics in the photoinduced non-equilibrium states. First, as RXD is directly sensitive to the long-range CO, the absence of the fastest dynamics, ~0.5 ps, suggests that this kinetics is linked to microscopic relaxation processes of non-equilibrium electronic states and is not directly linked to the restoration of long-ranged CO. Second, the similar timescales between and suggests that they likely share a common origin. As this dynamics is seen in both the local (average) charge distribution channel (Δ R/R ) and the long-range order channel (XRD), it is reasonable to attribute this dynamics to the recovery of the magnitude of the charge density modulation, that is, the CO order parameter's amplitude. Most interestingly, the recovery of the order parameter's amplitude does not occur simultaneously with the recovery of the CO diffraction peak intensity and indicates the importance of phase fluctuations in determining the recovery time of the CO itself. Phase fluctuations could be viewed as vibrations of the electronic lattice (that is, the periodic CO-related charge density modulation), analogous to vibrations of the crystal lattice. Although the exact functional form is somewhat debated, it has been demonstrated for charge density wave systems that fluctuations of the order parameter's phase can qualitatively give rise to a Debye–Waller suppression of the CO diffraction peaks in addition to the lattice Debye–Waller factor [20] , [21] , [22] . As the RXD signal is mostly sensitive to electronic CO scattering, only the phase Debye–Waller factor will be captured in our time-resolved XRD data. In accordance with our results, the slower component of the CO peak intensity recovery ( ) is most likely dominated by diminishing phase fluctuations of the CO order parameter. We note that phase fluctuation can be produced because the phase excitations are often gapless or acquire a small gap owing to pinning by the lattice or defects, and hence require little energy to excite. In addition, as the phase Debye–Waller factor exponentially suppresses the CO peak intensity scaling with the square of average phase fluctuation, small amounts of phase fluctuation can significantly suppress the CO peak intensity [20] . The interpretation of as due to phase fluctuation is also consistent with the fact that is much more sensitive to pump fluence ( Fig. 3c ), distinct from the other two timescales. From the presented evidence, is a direct measure of how fast energy can be transferred out of phase fluctuations and contains information about how strongly phase excitations (that is, phasons) couple to the lattice (that is, phonons). In the limit of zero excitation density, the phase fluctuation magnitude is infinitesimally small, thus can be thought to represent the intrinsic equilibration phason–phonon coupling timescale, τ φ −ph . By extrapolating to zero excitation density in Fig. 3b , we estimate τ φ −ph to be approximately 15 ps. We note that this is a lower bound of the phason-phonon relaxation timescale. Pinning effects introduced by disorder that limits the length scale of CO may also provide another mechanism for phason damping. High-voltage resistivity measurements suggest that these effects are non-negligible [29] . Nevertheless, τ φ −ph is more than one order of magnitude slower than the electron-phonon relaxation time, which is estimated to be ~0.4 ps by extrapolating to zero excitation density. This suggests that phason–lattice coupling is still much weaker than electron–phonon coupling. The dynamics of CO in the photo-excited transient state are summarized in Fig. 4a . At the earliest times in region I, the electronic energy abruptly increases due to the absorption of photons from the pump, causing the CO amplitude (Δ) suppression and generating phase ( τ φ −ph ) fluctuations. The excited electrons first decay rapidly, shedding energy, for example, into lattice relaxation (~0.5 ps), and the CO amplitude recovers on a timescale of ~2 ps. In region II, the amplitude of the CO order parameter has mostly recovered, but the phase continues to fluctuate, accounting for most of the remaining excited electronic energy. It is found that the timescale for equilibration between the phase fluctuations and the lattice is long (>15 ps), hence limiting the recovery. In addition, CO remains long ranged without changing its period in either region I or II; this indicates that whereas the photoinduced transient state involves the amplitude and phase fluctuations, topological defects are not created as they require reconfiguring a large number of spins and charges at a large energy cost. This is in stark contrast to the physics near the equilibrium phase transition temperature ( Fig. 4b ), where low-energy topological defects [28] reduce the correlation length and the amplitude of the CO order parameter. 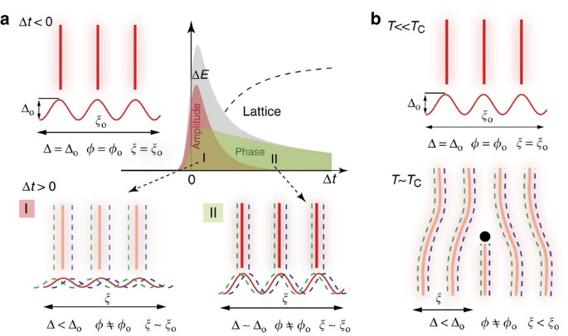Figure 4: Illustration of CO order parameter dynamics. (a) The photo-excited CO dynamics. ΔEis the energy difference with respect to the ground state energy. The grey shaded area represents the total ΔEin the long-ranged CO channel, whereas the red and green areas represent the ΔEcontribution of the amplitude and phase, respectively. The dissipation of ΔEthrough the coupling to the lattice degree of freedom results in the recovery of the CO order parameter and the increase of lattice energy, as indicated by the area below the black dashed line (labelled 'Lattice'). The order parameter completely recovers when the absorbed energy eventually dissipates entirely to the sample environment. Sketches of order parameters at three representative temporal regions are also shown. In each sketch, the red stripes illustrate the CO in real space (that is, the charge stripes) whose order parameter is symbolically drawn below as the red sinusoidal wave. The brightness of the stripe also represents the amplitude of the order parameter. The dashed sinusoidal waves and lines with green and blue colours illustrate the fluctuations of the phase of the CO order parameter. In these sketches, Δ,φandξ, respectively represent the amplitude, phase and the phase–phase correlation length of the CO order parameter. (b) Sketches for CO evolution in thermal equilibrium. Near the phase transition temperatureTC, in addition to the Gaussian phase fluctuation (green and blue dashed lines), large phase fluctuations also occur and create topological defects (black dot), reducing the coherence length and amplitude of the CO order parameter. Figure 4: Illustration of CO order parameter dynamics. ( a ) The photo-excited CO dynamics. Δ E is the energy difference with respect to the ground state energy. The grey shaded area represents the total Δ E in the long-ranged CO channel, whereas the red and green areas represent the Δ E contribution of the amplitude and phase, respectively. The dissipation of Δ E through the coupling to the lattice degree of freedom results in the recovery of the CO order parameter and the increase of lattice energy, as indicated by the area below the black dashed line (labelled 'Lattice'). The order parameter completely recovers when the absorbed energy eventually dissipates entirely to the sample environment. Sketches of order parameters at three representative temporal regions are also shown. In each sketch, the red stripes illustrate the CO in real space (that is, the charge stripes) whose order parameter is symbolically drawn below as the red sinusoidal wave. The brightness of the stripe also represents the amplitude of the order parameter. The dashed sinusoidal waves and lines with green and blue colours illustrate the fluctuations of the phase of the CO order parameter. In these sketches, Δ, φ and ξ , respectively represent the amplitude, phase and the phase–phase correlation length of the CO order parameter. ( b ) Sketches for CO evolution in thermal equilibrium. Near the phase transition temperature T C , in addition to the Gaussian phase fluctuation (green and blue dashed lines), large phase fluctuations also occur and create topological defects (black dot), reducing the coherence length and amplitude of the CO order parameter. Full size image Finally, we remark that the physics described in our study should be generally applicable to the recovery of complex order parameters in other systems, as long as the pump excitation density is not strong enough to excite defects in the phase ordering and when the phase modes are soft and couple weakly to the lattice. Photoinduced phase fluctuations may be crucial to understanding the mechanism of photoinduced superconductivity in the striped cuprates [2] . Materials Single crystals of La 1.75 Sr 0.25 NiO 4 were grown using the floating zone method. The crystals were first oriented using Laue diffraction and cut along the [1 0 0] surface. Orthorhombic notation was used to express the crystal structure where [1 0 0] is 45° to the Ni-O bond direction. The surface was then polished for experiments. The phase-transition temperature for CO is approximately 110 K. X-ray FEL configurations Experiments were performed at the SXR beamline 30 , LCLS, using the high-charge mode (250 pC, 70 fs) at a repetition rate of 60 Hz. The X-ray absorption spectrum (XAS) near the Ni L 3 -edge was first measured to calibrate the incident photon energy ( Supplementary Fig. S1a ). Then, the incident photon energy was tuned to the Ni-L 3 peak in XAS to perform resonant diffraction on SO and CO. The scattering geometry is sketched in Supplementary Fig. S1b . The chosen band width of approximately 1.6 eV covers the energy range of the primary resonance of the CO/SO diffraction peaks [15] , yielding the maximal intensity. The transverse beam spot on the sample was 300 μm×300 μm and the front-end N 2 gas attenuator (set at approximately 10–30% transmission) was used to avoid radiation damage from the LCLS beam. The average FEL pulse energy was 0.5 mJ per pulse. With an estimated photon band pass associated with the selected resolution (16%) and the combined beamline efficiency (2.5%), we estimated the FEL fluence on sample surface to be approximately 0.6 mJ cm −2 . The polarization of the FEL is in the scattering plane. Pump-probe configurations Photoexcitation was achieved via laser pulses with central wavelength at 800 nm from a Ti:sapphire laser amplifier system. Spatial overlap between the pump laser and X-ray FEL was achieved using the X-ray-induced fluorescence of an unpolished YAG crystal, viewed by three cameras from three different angles. To ensure a homogeneous excitation of the region probed by the X-ray FEL, the pump laser spot diameter (FWHM) was set at 720 μm, which is more than twice as large as the X-ray FEL spot. The pump fluence was varied with a combination of the neutral density filters and a wave plate and polarizer. The excitation density was estimated by taking into account the projected area on the sample surface corresponding to the angle of incidence, the absorption coefficient determined by reflectivity measurements and the optical penetration depth calculated from the measured complex index of refraction on the same sample ( Supplementary Fig. S2 and Supplementary Methods ). The direction of pump pulse polarization is the same as the X-ray FEL pulse, in the scattering plane. Coarse temporal overlap between the optical laser pump and the FEL-probe pulses was achieved by monitoring the photoelectric signal of the two beams when overlapped onto the tip of a coaxial cable inside the vacuum chamber. The signal from this coaxial cable was measured directly with a 13 GHz bandwidth oscilloscope. By matching the rising edges of the time traces from the two signals, the temporal overlap could be determined with <3 ps accuracy. Once coarse timing was established, the pump-probe delay time was varied with a mechanical delay stage. The fine temporal overlap was determined directly by monitoring the sample diffraction signal versus time delay. The time zero was defined to be the onset of pump-probe signal. The data were taken by randomly sampling the delay time within a given range. Data collection and process A compact fast-CCD (cFCCD), developed by the Engineering Division of Lawrence Berkeley Laboratory [19] , was used to record a two-dimensional cross section of the diffraction. It was mounted on an in-vacuum stage to allow the movement of the detector to cover almost the entire lower scattering hemisphere to image the diffraction peaks. The cFCCD has a maximum readout rate of 200 frames per second, allowing data acquisition on a pulse-by-pulse basis. The active area has a 240 (V) by 480 (H) array of 30 μm square pixels. At 100 mm away from sample, the detector pixel resolution was better than 0.02° and the effective acceptance angle was around 4° (V) by 8° (H). An image was collected for every LCLS pulse along with the encoder position of the mechanical delay stage and corresponding X-ray pulse information for that image. In particular, information of phase cavity that measures the arriving time of the electron bunch was also recorded to partially correct timing jitter between the pump laser and X-ray pulse [21] . After each data run, approximately 1,000 images were collected with the X-ray shutter closed and averaged together as a representative dark count image. This dark count image was subtracted from every image recorded in the associated data run. Because of small thermal drifts and fluctuations in the dark counts with time, an additional background adjustment was implemented for each shot using a small integrated region at the corner of the CCD image. The pump-probe delay time was calculated from the encoder position and phase cavity information. Then the images were binned and averaged according to the measured delay time. In addition, each image was also normalized by the incident photon flux ( I 0 ), which was measured through the photocurrent from an in-line aluminium foil. Because of the LCLS energy and intensity fluctuations, some of the images contained very weak signals due to low X-ray intensity while still having similar thermal noise inherent to the CCD array. Thus, an I 0 threshold was used to eliminate the images from the weaker LCLS pulses to maximize the signal-to-noise ratio. The I 0 threshold was set to eliminate approximately half of the collected images. The cFCCD has inherent gain and offset variations among the different active arrays, causing the stripe-like feature on the collected images. After the images were normalized, binned and averaged, a ten-pixel-wide region at the edge of the image, away from the peak, was used to generate an instrument transmission function. The image intensities were then adjusted according to this transmission function and were processed through a low pass filter to yield a smoother image. A region of interest was chosen to measure the integrated peak intensity from the processed average image representing the different delay times. We note that the integrated intensity is rather insensitive to the image processing we have applied. Optical pump-probe reflectivity measurement The ultrafast optical reflectivity change was measured by a pump-probe experimental set-up based on a femtosecond Ti:sapphire laser system. Ultrafast laser pulses at kilohertz repetition rate can be generated from this system with 100 fs pulse duration, 800 nm centre wavelength and 0.5 mJ per pulse energy. The pulses were split into pump and probe arm and then recombined onto the nickelate sample surface. The probe pulse reflected from the sample was detected by a photo-diode detector and its reflectivity change due to the pump pulse was measured by a standard lock-in detection scheme. The sample was kept in a closed-cycle helium cryostat, where the temperature can be controlled from room temperature to 20 K. The measurement geometry is similar to Supplementary Fig. S1b , except the angle of incident is approximately 5°. The polarization of the pump is in the plane of incidence ( b - c plane of the nickelate), whereas the polarization of probe is perpendicular to the plane of incidence ( a - b plane of the nickelate). How to cite this article: Lee, W. S. et al . Phase fluctuations and the absence of topological defects in a photo-excited charge-ordered nickelate. Nat. Commun. 3:838 doi: 10.1038/ncomms1837 (2012).